Mapping the 3D surface potential in Bi2Se3 Bi 2 Se 3 initially emerged as a particularly promising host of topological physics. However, in actual materials, several issues have been uncovered including strong surface band bending and potential fluctuations. To investigate these concerns, we study nominally stoichiometric Bi 2 Se 3 using scanning tunnelling microscopy. Here we identify two distinct distributions of Bi Se antisites that act as nanometer-scale sensors for the surface band-bending field. To confirm this, we examine bulk Cu-doped Bi 2 Se 3 and demonstrate a significantly reduced surface band-bending field. In addition, we find that in the case of unintentionally doped Bi 2 Se 3 , lateral fluctuations of the Dirac point can be directly correlated with specific near-surface point defects, namely Se vacancies. Bi 2 Se 3 has emerged as a particularly interesting host of topological physics due to its non-trivial surface state [1] , [2] , [3] . Initial studies indicated that theoretical predictions were largely true—topological protection reduces scattering and carriers are helical Dirac-like fermions [4] , [5] , [6] , [7] . However, further investigation raised several issues with its physical and structural properties in actual materials: Bi Se antisites may allow scattering from the surface to the bulk [8] , [9] , strong band bending creates an additional, topologically trivial, surface state [10] , [11] , [12] , [13] , and deep, unobservable charges may cause fluctuations in the Dirac point [4] . To address these concerns, we conducted scanning tunnelling microscopy (STM) studies on nominally stoichiometric Bi 2 Se 3 . We have identified two distinct Bi Se antisite distributions using spectroscopic imaging and ab initio simulations; their energy states are sensitive to the local valence band position and operate as depth-dependent potential sensors. Using these sensors, we generate nanometer-scale measurements of a strong surface band-bending (SBB) field that is tunable with bulk dopants, which we demonstrate with measurements on Cu x Bi 2 Se 3 . In addition by mapping the lateral fluctuations of the Dirac point with d I /d V imaging, we show spatial correlation of the potential fluctuations with specific near-surface point defects. Disparate influences are observed for different defects: Se vacancies cause Dirac point shifts, whereas Bi Se defects follow the Dirac point shifts. Band bending Early STM reports of the surface of Bi 2 Se 3 revealed two primary forms of native point defects: triangular topographic features and purely electronic defect states [14] . The triangular defects have been identified as Se vacancies, which n-dope the sample [15] , and are prominently visible in Fig. 1a . The second defect type is the Bi Se antisite (where a Bi atom replaces a Se lattice site) and is best observed near or below the Dirac point by d I /d V imaging ( Fig. 1b ), which provides a map proportional to the local density of states at a given bias. The peculiar features observed for Bi Se , like those shown in the atomic resolution topograph in Fig. 1c , has led some recent studies to attribute them to surface-bulk scattering near the Dirac point [8] —however, angle-resolved photoemission spectroscopy (ARPES) results have not observed a side lobe to the valence band, necessary for this interpretation, and the feature geometry does not change at different biases ( Supplementary Figs S1 and S2 ), which is inconsistent with the proposed scattering states. We therefore attribute the defect features to impurity states unassociated with bulk-surface scattering. 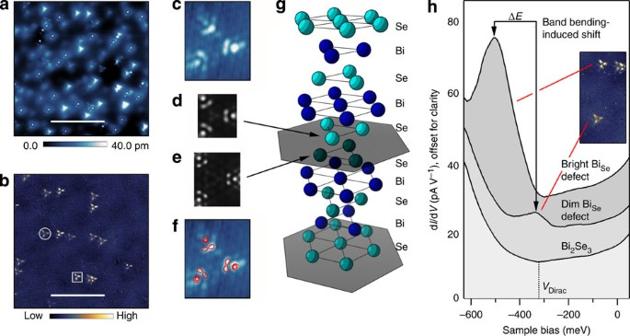Figure 1: Topographic and spectroscopic identification of BiSedefects. (a) Topography showing Se vacancies and corresponding dI/dVimage (b) showing BiSedefects in Bi2Se3at −380 meV,I=500 pA. (c) 2.9 × 3.5 nm atomic resolution imaging of a BiSedefect at −500 meV andab initioSTM simulations for a BiSedefect in the 5th (d) and 6th (e) layer at the same scale. (f) Contours fromdoverlaid onc. (g) Atomic structure of Bi2Se3, where hexagons separate the quintuple layers. (h) dI/dVspectroscopy on two defect types, taken on their lobes: the dim defect type, labelled with a circle inb, and a bright defect type, labelled with a square inb, as well as spectroscopy taken away from any defects. The bright and dim defects show a significant difference in their energy position on undoped Bi2Se3. To physically distinguish the defects, the lobes on the dim defects are slightly further from the centre, more likely corresponding to a deeper defect as per the simulation ine, whereas the bright defect is more compact, better corresponding tod. The scale bar inaandbis 30 nm. Figure 1: Topographic and spectroscopic identification of Bi Se defects. ( a ) Topography showing Se vacancies and corresponding d I/ d V image ( b ) showing Bi Se defects in Bi 2 Se 3 at −380 meV, I =500 pA. ( c ) 2.9 × 3.5 nm atomic resolution imaging of a Bi Se defect at −500 meV and ab initio STM simulations for a Bi Se defect in the 5th ( d ) and 6th ( e ) layer at the same scale. ( f ) Contours from d overlaid on c . ( g ) Atomic structure of Bi 2 Se 3 , where hexagons separate the quintuple layers. ( h ) d I/ d V spectroscopy on two defect types, taken on their lobes: the dim defect type, labelled with a circle in b , and a bright defect type, labelled with a square in b , as well as spectroscopy taken away from any defects. The bright and dim defects show a significant difference in their energy position on undoped Bi 2 Se 3 . To physically distinguish the defects, the lobes on the dim defects are slightly further from the centre, more likely corresponding to a deeper defect as per the simulation in e , whereas the bright defect is more compact, better corresponding to d . The scale bar in a and b is 30 nm. Full size image We observed that Bi Se defects show tunnelling amplitude maxima at vastly different voltages—for example, Fig. 1h shows d I /d V spectroscopy for two defects whose tunnelling maxima are separated by ~150 meV. By analyzing the d I /d V spectra from numerous Bi Se defects, a histogram analysis shows that there is a bimodal distribution ( Fig. 2a ). Therefore, contrary to previous reports [14] , these nearly identical features are due to Bi Se defects at two separate Se layers. From ab initio calculations, we can rule out the middle layer (Bi Se2 ) due to its high energy of formation [16] , which means that the defects are in structurally equivalent locations (that is, the top or bottom of a quintuple layer—these positions are symmetric). Structurally equivalent defects at different depths should be energetically degenerate. However, in this case, the degeneracy is broken by surface band-bending mapping the defect energies at different depths maps the local band bending. On the basis of our ab initio simulations of STM topographs for these defects ( Fig. 1d,e ), we attribute the higher amplitude defect (square in Fig. 1b ) to Bi Se on the 5th layer and the lower amplitude defect (circle in Fig. 1b ) to Bi Se on the 6th atomic layer, which correspond to the bottom of the 1st quintuple layer and the top of the 2nd quintuple layer, respectively (see Fig. 1g and Supplementary Fig. S3 ). The n-shifted defect has a higher tunnelling amplitude, meaning that it is closer to the surface/STM tip, demonstrating downward SBB of the bulk conduction and valence bands. Downward SBB is consistent with ARPES observations [10] , and is possibly due to more Se vacancies forming at the sample–vacuum interface following the ultra high vacuum (UHV) sample cleave. 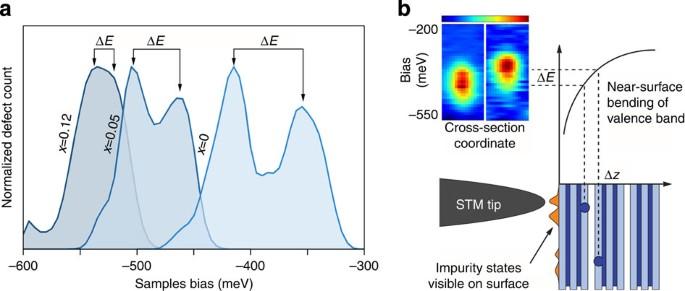Figure 2: Defect distributions and detecting near-surface band bending. (a) Histograms of the BiSedefect energies in CuxBi2Se3, extracted from multipass dI/dVimages, show a decreasing gap between the peaks as the Cu content is increased. (b) Schematic of the proposed band-bending mechanism responsible for the energy difference between the defects; the orange profile represents the BiSedefect’s observable states on the Bi2Se3surface. Cross-sectional dI/dVlinescans from two different defects on Bi2Se3are shown for direct comparison, as well. Colour scale ranges inb: left, 1.4 × 10−11pA meV−1, right, 5.0 × 10−12pA meV−1. Figure 2: Defect distributions and detecting near-surface band bending. ( a ) Histograms of the Bi Se defect energies in Cu x Bi 2 Se 3 , extracted from multipass d I/ d V images, show a decreasing gap between the peaks as the Cu content is increased. ( b ) Schematic of the proposed band-bending mechanism responsible for the energy difference between the defects; the orange profile represents the Bi Se defect’s observable states on the Bi 2 Se 3 surface. Cross-sectional d I/ d V linescans from two different defects on Bi 2 Se 3 are shown for direct comparison, as well. Colour scale ranges in b : left, 1.4 × 10 −11 pA meV −1 , right, 5.0 × 10 −12 pA meV −1 . Full size image These defects should retain their position relative to the valence band, so adding an n-type dopant, like incorporating Cu into the bulk, should n-shift the entire electronic structure including the Bi Se distributions, without altering the nature of the Bi Se defect itself (see Supplementary Fig. S4 for more information). We have observed several sub-surface Cu defect types in the topography ( Fig. 3a ), but they do not appear to have changed the shape of the Bi Se defects in a significant way, as shown in the d I/ d V images in Fig. 3b–f . The identification of these Cu defects varies in the literature [17] , [18] , so the implications of their structural configurations within the lattice are left to future studies. Regardless of the defects’ identities, the observed Cu defect density does not suggest that significant structural changes have occurred, allowing us to consider them, simply, as dopants. Upon adding Cu, we observed the two Bi Se distributions shift closer together ( Fig. 2a ). From the band-bending picture, this means that the SBB is reduced ( Fig. 2b ). As more carriers are introduced with higher n-type doping (more of the bulk conduction band is below the Fermi level), we believe screening effects are causing the reduction in the band-bending potential field. 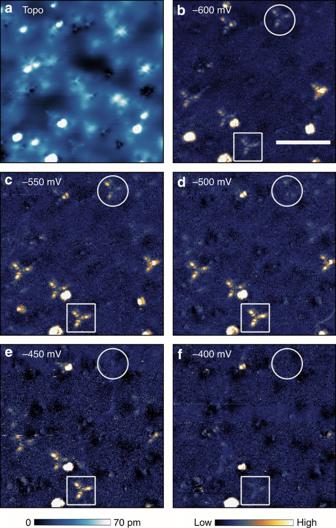Figure 3: Cu defects in Bi2Se3. Cu doping introduces a number of new defects, as shown in the topograph ina. However, as shown in the dI/dVdata inb–f, the distinct BiSedefect is still present. Indeed, it still shows up at different biases depending on its layer, as highlighted by the circled and squared defects. Scale bar inbis 10 nm. Figure 3: Cu defects in Bi 2 Se 3 . Cu doping introduces a number of new defects, as shown in the topograph in a . However, as shown in the d I/ d V data in b – f , the distinct Bi Se defect is still present. Indeed, it still shows up at different biases depending on its layer, as highlighted by the circled and squared defects. Scale bar in b is 10 nm. Full size image We have considered the possibility that the band bending was induced by the electric field from the STM tip, an effect known as tip-induced band bending (TIBB). We performed spatial spectroscopic imaging at a variety of tunnelling set points (150–500 pA) and observed less than a 5-meV shift in the impurity peak position ( Supplementary Fig. S5 ), indicating that TIBB is not the dominant source of the energy shift. Presumably, as the surface is already n-doped even in the case of zero Cu doping, the available free carrier concentration is high enough to screen out the tip-induced field. To quantitatively approximate the magnitude of SBB as a function of doping ( Fig. 4a ), the energy separation of the defect distributions is divided by the approximate separation between the Se layers terminating adjacent quintuple layers, as determined by local-density approximation energy relaxation calculations. We note that intercalation of Cu increases the separation between layers [18] , and any TIBB effects would further amplify the observed bending. Therefore, the values we have measured are upper bounds. 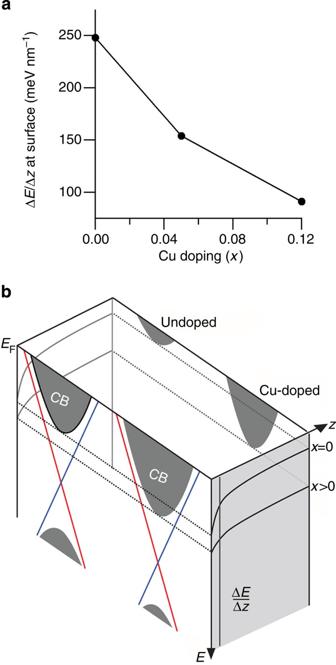Figure 4: Influence of Cu doping on the surface potential. (a) Band bending as a function of doping level. To numerically determine the band bending, we used the distance determined byab initiosimulations of 0.254 nm. (b) Schematic showing the surface potential dependence on doping. In Cu-doped samples, more of the bulk conduction band is below the Fermi energy, providing enough carriers to screen the band bending. Figure 4: Influence of Cu doping on the surface potential. ( a ) Band bending as a function of doping level. To numerically determine the band bending, we used the distance determined by ab initio simulations of 0.254 nm. ( b ) Schematic showing the surface potential dependence on doping. In Cu-doped samples, more of the bulk conduction band is below the Fermi energy, providing enough carriers to screen the band bending. Full size image Several groups have observed bulk two-dimensional electron gas (2DEG) states appearing on samples left in vacuum, and the ARPES data suggest band bending is the culprit [10] , [11] , [12] , [13] . STM is surface sensitive, so this calls into question the results of all STM studies above the conduction band minimum on this material: is the measured surface state really of topological origin, or simply due to a traditional bulk 2DEG? If a 2DEG exists, it can be eliminated by reducing the SBB. To ensure that future STM studies are truly investigating the topological surface state in Bi 2 Se 3 , control of the surface potential will be essential—bulk n-type doping provides one such mechanism, as shown schematically in Fig. 4b . Correlating potential fluctuations The Dirac point shifts rigidly with bulk band fluctuations [4] ( Fig. 5a ) and the d I /d V data ~200 meV below the Dirac point are effectively linear with bias, allowing us to map the d I /d V value below the Dirac point to the fluctuations of the Dirac point. This technique has been successfully applied to graphene [19] , and we confirmed the validity of this technique for Bi 2 Se 3 from line spectroscopy data, as shown in Fig. 5b,c . However, d I /d V images can contain additional information that could be interpreted as quasiparticle scattering [20] or variations in the apparent barrier height [21] , so we quantitatively demonstrated that above the Dirac point ( Fig. 5f ), the d I /d V image is a reversal of the d I/ d V image below Dirac point with a cross-correlation coefficient of −0.5. Therefore, the d I/ d V images in Fig. 5d,e are best described as maps of Dirac point shifts. 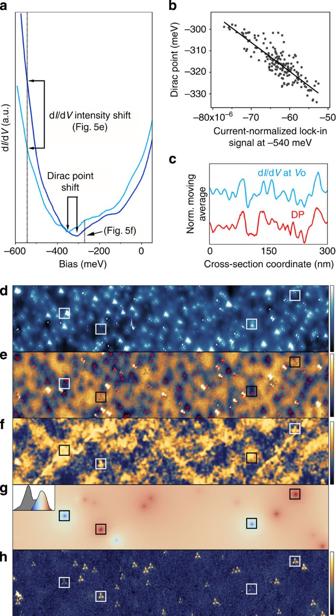Figure 5: Correlating potential fluctuations with point defects. (a) Two dI/dVcurves taken from different regions on Bi2Se3show how the Dirac point shift can be correlated, to first order, with the intensity shift in dI/dVintensity—this allows single-pass dI/dVscans to map the Dirac point fluctuations. (b) A scatter plot determined from line spectroscopy data across 300 nm of Bi2Se3shows the first-order relation between the Dirac point and the lock-in signal at −540 meV;R2=0.72. (c) Seven-point moving average from the line spectroscopy visually shows the correlation fromb. A 350 × 50 nm region of Bi2Se3is then investigated with this technique: topography (d) at −200 meV shows Se vacancies, and the dI/dVimage of the same region taken at −540 meV shows fluctuations in the Dirac point (e). Ine, the red circles represent bright triangular defects, determined fromd. (f) dI/dVimage at −270 meV showing that the dI/dVmap gives an inverse image ofeabove the Dirac point. The cross-correlation coefficient is −0.5, quantitatively confirming the contrast reversal despite the higher noise level inf. A visualization of the deviations from the distribution mean for dim-type BiSedefects is shown ing, where red points indicate a BiSedefect with an energy state that is more positive than the distribution mean, and blue points indicate a BiSedefect below the distribution mean (see inset). The dI/dVimage at −350 meV (h) shows both dim and bright type defects. The fluctuations in the BiSedefect energy scale correlates directly with the fluctuations in the Dirac point; a few extreme examples are highlighted in boxes ine–h. Colour scales:d, 40 pm;e, 30 meV;h, 10 pA/V. Figure 5: Correlating potential fluctuations with point defects. ( a ) Two d I/ d V curves taken from different regions on Bi 2 Se 3 show how the Dirac point shift can be correlated, to first order, with the intensity shift in d I/ d V intensity—this allows single-pass d I/ d V scans to map the Dirac point fluctuations. ( b ) A scatter plot determined from line spectroscopy data across 300 nm of Bi 2 Se 3 shows the first-order relation between the Dirac point and the lock-in signal at −540 meV; R 2 =0.72. ( c ) Seven-point moving average from the line spectroscopy visually shows the correlation from b . A 350 × 50 nm region of Bi 2 Se 3 is then investigated with this technique: topography ( d ) at −200 meV shows Se vacancies, and the d I/ d V image of the same region taken at −540 meV shows fluctuations in the Dirac point ( e ). In e , the red circles represent bright triangular defects, determined from d . ( f ) d I /d V image at −270 meV showing that the d I/ d V map gives an inverse image of e above the Dirac point. The cross-correlation coefficient is −0.5, quantitatively confirming the contrast reversal despite the higher noise level in f . A visualization of the deviations from the distribution mean for dim-type Bi Se defects is shown in g , where red points indicate a Bi Se defect with an energy state that is more positive than the distribution mean, and blue points indicate a Bi Se defect below the distribution mean (see inset). The d I/ d V image at −350 meV ( h ) shows both dim and bright type defects. The fluctuations in the Bi Se defect energy scale correlates directly with the fluctuations in the Dirac point; a few extreme examples are highlighted in boxes in e – h . Colour scales: d , 40 pm; e , 30 meV; h , 10 pA/V. Full size image Figure 5d and e shows the topography and corresponding map of Dirac point fluctuations, respectively, in nominally stoichiometric Bi 2 Se 3 . Se vacancies observed in Fig. 5d , indicated with red circles in Fig. 5e , can be correlated with n-shifts in the Dirac point. The energy of formation for Se vacancies increases as the sample is n-doped [16] —so they would preferentially form in more positively shifted regions. Therefore, their correlation with negatively shifted regions suggests they are causing the n-type fluctuations. It is also apparent that these defects are the origin of the fluctuations (responsible for the finite width of the peak energy distributions in Fig. 2a ) in the Bi Se distributions: negatively shifted Bi Se defects are on negatively shifted regions of the sample and positively shifted Bi Se defects are found on positively shifted regions of the sample ( Fig. 5e–h ). Significantly, while these Bi Se defects do have strong electronic interactions, they do not appear to have strong effects on the position of the Dirac point, rather, they appear to follow the bulk fluctuations. Our re-evaluation of the Bi Se defect as an impurity state suggests that bulk-surface interactions are not directly evident. Furthermore, this classification allows the band bending to be directly visualized, highlighting the concerns that non-topological surface states may be inadvertently formed on Bi 2 Se 3 . To prevent the formation of such a state, it will be important to deliberately tailor the band bending using advanced synthesis techniques such as molecular beam epitaxy. Furthermore, by correlating observable defects with the fluctuations in the Dirac point through d I /d V imaging, we have shown that different defects influence the Dirac point disparately—as different preparation techniques produce different characteristic defects, an understanding of the interplay between specific defects and the local electronic structure is critical. We expect that such atomic-scale insights will enable application-optimal doping and growth schemes. Ultimately, Bi 2 Se 3 remains a model system for exploring topological physics. Sample growth Ternary Cu x Bi 2 Se 3 bulk crystals were grown by the vertical Bridgman technique using a three-zone high-temperature furnace. The temperature profiles in the growth zone were designed to produce a 3–5 °C axial gradient. The starting materials used for crystal growth (6 N Bi and 6 N Se) were deoxidized and outgassed under vacuum directly before use. Stoichiometric amounts of Bi and Se along with 6 N purity deoxidized Cu were enclosed in a graphitized fused quartz ampoule, evacuated for several hours and sealed off under a dynamic vacuum of ~10 −8 torr. The pre-loaded charge was then placed in the middle zone of the furnace. After the preliminary reaction was completed at 400 °C, the charge was slowly heated up to 770 °C for ~6 h and then the melt was allowed to homogenize for 24 h under a high linear temperature gradient to promote mixing. The melt was solidified with a rate of about 1.5 mm h −1 at a small linear gradient of 3–5 °C cm −1 . Ab initio calculations Our calculations are based on density functional theory with the Perdew-Burke-Ernzerhof approximation [22] . Interactions between ion cores and valence electrons are described by the projector augmented wave method [23] , [24] , as implemented in the VASP package [25] , [26] . Plane-waves with a kinetic energy cutoff of 270 eV were used as the basis set. We used a (7 × 7) double quintuple slab containing 196 Bi and 294 Se atoms with gamma point sampling of the Brillouin zone. All atoms were allowed to relax with a convergence criterion for the structural relaxations of 0.04 eV Å −1 . To compare with experiment, we simulate the STM images based on the theory of Tersoff and Hamann [27] . When simulating STM images for comparison with experimental images, care has to be taken with regard to the location of the experimental Fermi energy. To correspond to the observed images at a −500 meV bias, the Fermi energy window used to construct the charge density for the simulated images range from conduction band minimum +300 meV to the valence band maximum +100 meV. This window is chosen relative to the band edges because the use of only two slabs increases the theoretical gap. STM measurements Samples were cleaved in an UHV with a base pressure <10 −10 torr, then immediately transferred to the STM at liquid nitrogen temperature. The STM is a Pan-type STM scan head from RHK in a home-built UHV chamber. Electrochemically etched tungsten STM tips were cleaned by e-beam irradiation under UHV. STS data were taken using the built-in lock-in amplifier on a Nanonis STM controller at 780 Hz and 10-mV modulation amplitude. STM topographs were taken in constant current mode and the bias was applied to the sample. Bi Se peak positions were determined from multipass scan data at constant current, unless otherwise noted, and were extracted from the lobes of the defects; the background spectra, averaged on either side of the given lobes, were subtracted from the impurity peak spectra to remove systematic offsets due to the shape of the nearby d I/ d V spectra. More information is provided with Supplementary Fig. S6 . How to cite this article: Mann, C. et al. Mapping the 3D surface potential in Bi 2 Se 3 . Nat. Commun. 4:2277 doi: 10.1038/ncomms3277 (2013).